Receptor tyrosine kinase c-Met controls the cytoskeleton from different endosomes via different pathways Receptor tyrosine kinases (RTKs) are increasingly recognized as having the capacity to signal post-internalization. Signalling outputs and/or duration, and subsequent cellular outcome, are thought to be distinct when emanating from endosomes compared with those from the plasma membrane. Here we show, in invasive, basal-like human breast cell models, that different mechanisms are engaged by the RTK c-Met in two different endosomes to control the actin cytoskeleton via the key migratory signal output Rac1. Despite an acute activation of Rac1 from peripheral endosomes (PEs), c-Met needs to traffic to a perinuclear endosome (PNE) to sustain Rac1 signalling, trigger optimal membrane ruffling, cell migration and invasion. Unexpectedly, in the PNE but not in the PE, PI3K and the Rac-GEF Vav2 are required. Thus we describe a novel endosomal signalling mechanism whereby one signal output, Rac1, is stimulated through distinct pathways by the same RTK depending on which endosome it is localized to in the cell. Endocytosis no longer is considered solely a desensitization mechanism and several receptors remain competent to signal on endosomes prior to their degradation [1] , [2] , [3] , [4] , [5] , [6] . The signalling outputs from endosomal receptors and subsequent cellular outcomes, including cell transformation and tumorigenesis, are thought to be distinct from those outputs triggered from the plasma membrane (PM) [7] , [8] , [9] , [10] . While this PM–endosome relationship is an accepted distinction, there is limited understanding of the signal outputs from different endosomal compartments, which have been considered principally to play roles in the sorting of receptors for downregulation or recycling. Receptors are able to signal from different endosomes, including the late endosome [7] . Nevertheless, signalling of a given receptor on a specific endosome generally has been compared with signalling from the PM. Whether a receptor can signal differently from distinct intracellular compartments and how this might influence cell behaviour is unknown. The receptor tyrosine kinase (RTK) and proto-oncogene c-Met clathrin and dynamin-dependent [10] , [11] endocytosis have been reported in several cell systems including MDCK [12] , [13] and HeLa cells [11] , [14] . c-Met endosomal signalling is required for full activation of ERK1/2 (ref. 15) [15] , its correct delivery to the PM and STAT3 nuclear accumulation [15] , [16] . These endosomal signalling capabilities are required for cell migration, consistent with other studies [9] , [17] , [18] . One key pathway controlling cell migration involves Rac1, a member of the Rho GTPase family, acting downstream of c-Met [19] , [20] , [21] , [22] . Generally, it has been accepted that Rac1 needs to be recruited to the PM to be activated [23] , [24] . However, a recent study, performed on HeLa cells, reported that, upon HGF stimulation, Rac1 is activated on endosomes before arriving at the PM where it triggers actin cytoskeleton dynamics necessary for cell migration [9] . This raises the questions as to where c-Met is localized during these processes. A critical stage in breast cancer, leading to poor outcome, is the transition of pre-invasive to invasive disease. c-Met and its ligand, hepatocyte growth factor (HGF), also called scatter factor, promote breast cancer cell motility, invasion [25] and in vivo tumorigenesis and metastasis [26] , [27] , [28] , [29] , [30] . c-Met is overexpressed in 20–30% of breast cancer cases [31] , correlating with a high risk of metastasis and poor prognosis [32] , [33] , [34] . It is upregulated in triple negative/basal tumours (oestrogen, progesterone, ErbB2 negative) and, in erbB2-positive tumours, is associated with poor outcomes [35] , [36] , [37] , [38] , [39] . It may contribute to trastuzumab [40] and gefitinib [41] resistance in ErbB2 or epidermal growth factor receptor (EGFR)-positive breast cancer. c-Met therefore has emerged as a therapeutic target and a possible independent prognostic factor [33] , [34] , [42] . Understanding the signalling mechanisms of c-Met in breast cancer may offer new opportunities in designing novel therapies. Here, we show that, to stimulate the migration of an invasive breast cancer model, HGF-activated c-Met sustains the Rac1 pathway from a perinuclear endosome (PNE) through the engagement of the specific effectors PI3K and Vav2. These intermediates, however, are not required for acute c-Met activation of Rac1 from peripheral endosome (PE). Thus, we report a novel endosomal signalling mechanism whereby one signal output, Rac1, is stimulated through distinct pathways by the same RTK depending on which endosome it is localized to in the cell. c-Met activates Rac1 post endocytosis in MDA-468 cells HGF stimulation for 10 and 30 min triggered Rac1 activation ( Fig. 1a ) and time-dependent Rac1 accumulation at the free edges of MDA-468 cells (31% of cells with PM Rac1 at 10 min and 48% at 30 min ( Fig. 1b ). This response was abrogated in cells pretreated with the c-Met tyrosine kinase inhibitor SU11274 ( Supplementary Fig. 1a ). In parallel to Rac1 activation, HGF stimulated a robust, time-dependent actin cytoskeleton rearrangement with a loss of stress fibres and an increase of cortical actin and membrane ruffling (29 and 46% of cells with membrane ruffles at 10 and 30 min, respectively) ( Fig. 1c ). Knocking down Rac1 by small interfering RNAs (siRNAs) prevented the HGF-dependent cytoskeleton rearrangement ( Supplementary Fig. 1b,c ). Thus, HGF stimulates membrane ruffling in MDA-468 cells through the activation of Rac1. 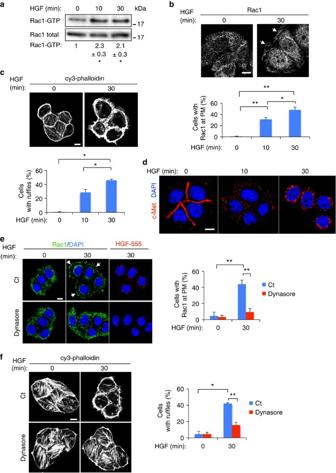Figure 1: c-Met activates Rac1 post endocytosis in MDA-468 cells. (a) Detection of Rac1-GTP with a GST-CRIB assay in cells stimulated with HGF for 0, 10 and 30 min. Below, the fold increase over non-treated cells. Data are presented as means±s.e.m. (n=3, *P<0.05, Student’st-test). (b) Confocal sections of cells stained for Rac1 in basal conditions and after HGF stimulation for 0 and 30 min. Scale bar, 10 μm. Arrows indicate Rac1 at the PM. The graph represents the percentage of cells with Rac1 at the PM. Data are presented as means±s.e.m. (n=4, *P<0.05 and **P<0.01, Student’st-test). (c) Confocal sections of cells stained with cyanin3-phalloidin in basal conditions and after HGF stimulation. Scale bar, 10 μm. The graph represents the percentage of cells with membrane ruffles. Data are presented as means±s.e.m. (n=3, *P<0.05, Student’st-test). (d) Confocal sections of cells stimulated with HGF for 0, 10 and 30 min and stained for c-Met (red) and DAPI (blue). Scale bar, 10 μm. (e) Confocal sections of cells stained for Rac1 (green) and DAPI (blue). Cells were starved for 24 h, pretreated or not with dynasore and stimulated with Alexa Fluor 555-conjugated HGF (HGF-555). Scale bar, 10 μm. The graph shows the percentage of cells with Rac1 at the PM. Data are presented as means±s.e.m. (n=3, **P<0.01, Student’st-test). (f) Confocal sections of cells stained with cyanin3-phalloidin in basal conditions and after 30 min of HGF stimulation with or without dynasore pretreatment. Scale bar, 10 μm. The graph shows the percentage of cells with membrane ruffles. Data are presented as means±s.e.m. (n=3, *P<0.05 and **P<0.01, Student’st-test). Figure 1: c-Met activates Rac1 post endocytosis in MDA-468 cells. ( a ) Detection of Rac1-GTP with a GST-CRIB assay in cells stimulated with HGF for 0, 10 and 30 min. Below, the fold increase over non-treated cells. Data are presented as means±s.e.m. ( n =3, * P <0.05, Student’s t -test). ( b ) Confocal sections of cells stained for Rac1 in basal conditions and after HGF stimulation for 0 and 30 min. Scale bar, 10 μm. Arrows indicate Rac1 at the PM. The graph represents the percentage of cells with Rac1 at the PM. Data are presented as means±s.e.m. ( n =4, * P <0.05 and ** P <0.01, Student’s t -test). ( c ) Confocal sections of cells stained with cyanin3-phalloidin in basal conditions and after HGF stimulation. Scale bar, 10 μm. The graph represents the percentage of cells with membrane ruffles. Data are presented as means±s.e.m. ( n =3, * P <0.05, Student’s t -test). ( d ) Confocal sections of cells stimulated with HGF for 0, 10 and 30 min and stained for c-Met (red) and DAPI (blue). Scale bar, 10 μm. ( e ) Confocal sections of cells stained for Rac1 (green) and DAPI (blue). Cells were starved for 24 h, pretreated or not with dynasore and stimulated with Alexa Fluor 555-conjugated HGF (HGF-555). Scale bar, 10 μm. The graph shows the percentage of cells with Rac1 at the PM. Data are presented as means±s.e.m. ( n =3, ** P <0.01, Student’s t -test). ( f ) Confocal sections of cells stained with cyanin3-phalloidin in basal conditions and after 30 min of HGF stimulation with or without dynasore pretreatment. Scale bar, 10 μm. The graph shows the percentage of cells with membrane ruffles. Data are presented as means±s.e.m. ( n =3, * P <0.05 and ** P <0.01, Student’s t -test). Full size image We then analysed c-Met localization using confocal microscopy. In unstimulated cells, c-Met is expressed at the PM. HGF binding led to a rapid internalization of c-Met. Thus at 10 min, c-Met was mostly detected in peripheral vesicles ( Fig. 1d ). This internalization is further illustrated by live confocal imaging of cells that have been preincubated on ice with Alexa Fluor 555-conjugated HGF (HGF-555) before imaging at 37 °C ( Supplementary Movie 1 ). It was verified that in MDA-468 cells, HGF-555 internalizes with c-Met ( Supplementary Fig. 1d ) [16] . c-Met trafficked further upon time and was more accumulated around the nucleus at 30 min ( Fig. 1d ). Perturbation of the endocytic machinery through pretreating the cells with dynasore, a cell-permeable inhibitor of dynamin [16] , [43] , which blocked HGF-555 uptake ( Fig. 1e right hand panels), inhibited HGF-dependent Rac1 activation ( Supplementary Fig. 2a ) and its localization at the free edges of cells ( Fig. 1e ). However, a post-internalization treatment (at 10 or 30 min) had no effect, excluding a direct influence of dynasore on the post-internalization activation or on the exocytic machinery responsible for the delivery of Rac1 to the PM ( Supplementary Fig. 2b,c ). Dynasore pretreatment also inhibited the HGF-dependent actin cytoskeleton rearrangement leading to a strong reduction in membrane ruffle formation ( Fig. 1f ). Finally, reduction of clathrin heavy chain expression through siRNA knockdown, which reduced c-Met internalization [16] , also reduced HGF-dependent Rac1 activation ( Supplementary Fig. 2d ) and HGF-dependent cell migration ( Supplementary Fig. 2e ). These results show that the endocytosis machinery is required for the stimulation of Rac1 by HGF, for the subsequent formation of ruffles and the migration of the invasive, basal-like human breast cell line MDA-468. They are consistent with the previously described discovery of active Rac1 on endosomes and subsequent influence on the reorganization of the actin cytoskeleton [9] , [10] . c-Met traffic to the PNE promotes optimal Rac1 activation As shown in Fig. 1 , 10 min of HGF stimulation triggered significant Rac1 activation, accumulation at the PM and membrane ruffle formation, suggesting that c-Met initially can trigger these responses from peripheral endosomes (PEs). However, a significant increase in the percentage of cells with Rac1 at the PM and membrane ruffling was detected at 30 min compared with 10 min of HGF stimulation, suggesting the perinuclear localization provides some additional/cumulative effect. In order to characterize the endosomal compartments at 10 and 30 min, GFP-fusions of Rab5, Rab4, Rab11 and Rab7 were expressed at low levels and the localization of c-Met or Alexa Fluor 555-conjugated HGF (HGF-555) uptake with each Rab was analysed by confocal microscopy. Although colocalization was detected with each Rab at both times, the proportions differed ( Fig. 2c ). At 10 min, HGF-555 colocalized mainly with GFP-Rab5 and GFP-Rab4 ( Supplementary Fig. 3a ). Interestingly, an increased overlap with the late endosomal marker GFP-Rab7 was observed at 30 min compared with 10 min ( Fig. 2a , Supplementary Fig. 3b,c , Supplementary Movie 2 , left hand panel). Thus the colocalization between c-Met bound HGF-555 and GFP-Rab7 increased significantly from 17% at 10 min to 42% at 30 min of stimulation ( Fig. 2a ). Consistent with this, the proportion of c-Met colocalizing with GFP-Rab7 over the colocalization with the other Rabs increased from 17% at 10 min to 33% at 30 min, thus corresponding to an enrichment of nearly twofolds. This represented the greatest enrichment as compared with Rab11 (1.3-fold increase) ( Supplementary Fig. 3d,e ) while at 30 min c-Met was decreased in Rab5 and Rab4 endosomes (by 0.8- and 0.7–fold, respectively) ( Fig. 2c ). Finally c-Met colocalized with the late endosomal marker Lamp1 at 30 min of HGF stimulation ( Supplementary Fig. 3f ). 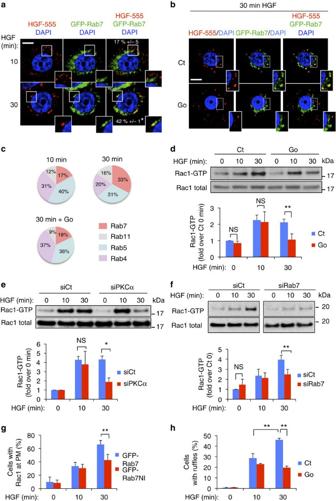Figure 2: c-Met traffic to the PNE promotes optimal Rac1 activation in MDA-468 cells. (a) Confocal sections of cells transfected with GFP-Rab7, stimulated with Alexa Fluor 555-conjugated HGF (HGF-555) (red) for 10 and 30 min and stained for DAPI (blue). Scale bar, 10 μm. The percentage of colocalization between HGF-555 and Rab7 at 10 and 30 min are indicated on the merged pictures. Data are presented as means±s.e.m. (n=3, *P<0.05, Student’st-test). The bottom panel is a magnification of the picture shown inSupplementary Fig. 3b. (b) Confocal sections of GFP-Rab7 transfected cells stimulated with HGF-555, pretreated for 20 min or not with the PKCα inhibitor Gö6976 (Go) and stained for DAPI (blue). Scale bar, 10 μm. (c) GFP-Rab(4, 5, 7, 11) transfected cells were stimulated with HGF-555 for 10 and 30 min, pretreated or not with PKCα inhibitor Gö6976 (Go) and colocalizations between HGF-555 and different Rabs proteins were quantified. The graphs represent the proportion of HGF-555 in Rab4, Rab5, Rab7 and Rab11 compartment. (d) Lysates from cells stimulated with HGF for times indicated, pretreated for 20 min or not with Gö6976. The lysates were subjected to a GST-CRIB pull-down assay. The graph shows the fold increases over control 0 min. Data are presented as means±s.e.m. (n=3, **P<0.01 and NS: nonsignificant, Student’st-test). (e) Lysates from cells transfected with control or PKCα siRNA and stimulated with HGF for the times indicated. The lysates were subjected to a GST-CRIB pull-down assay. The graph shows the fold increases over 0 min. Data are presented as means±s.e.m. (n=3, *P<0.05 and NS: nonsignificant, Student’st-test). (f) Lysates from cells transfected with control or Rab7 siRNA and stimulated with HGF for the times indicated. The lysates were subjected to a GST-CRIB pull-down assay. The graph shows the fold increases over Ct 0 min. Data are presented as means±s.e.m. (n=3, **P<0.01 and NS: nonsignificant, Student’st-test). (g) Percentage of cells with Rac1 at the PM. Data are presented as means±s.e.m. (n=5, **P<0.01, Student’st-test). Cells were transfected with a GFP-Rab7wt or GFP-Rab7NI, stimulated with HGF for 10 and 30 min, fixed and stained for Rac1. (h) Percentage of cells with ruffles. Data are presented as means±s.e.m. (n=3, **P<0.01, Student’st-test). Cells were pretreated or not for 20 min with Gö6976 (Go) and stimulated with HGF as indicated, fixed and stained with cyanin3-phalloidin. Figure 2: c-Met traffic to the PNE promotes optimal Rac1 activation in MDA-468 cells. ( a ) Confocal sections of cells transfected with GFP-Rab7, stimulated with Alexa Fluor 555-conjugated HGF (HGF-555) (red) for 10 and 30 min and stained for DAPI (blue). Scale bar, 10 μm. The percentage of colocalization between HGF-555 and Rab7 at 10 and 30 min are indicated on the merged pictures. Data are presented as means±s.e.m. ( n =3, * P <0.05, Student’s t -test). The bottom panel is a magnification of the picture shown in Supplementary Fig. 3b . ( b ) Confocal sections of GFP-Rab7 transfected cells stimulated with HGF-555, pretreated for 20 min or not with the PKCα inhibitor Gö6976 (Go) and stained for DAPI (blue). Scale bar, 10 μm. ( c ) GFP-Rab(4, 5, 7, 11) transfected cells were stimulated with HGF-555 for 10 and 30 min, pretreated or not with PKCα inhibitor Gö6976 (Go) and colocalizations between HGF-555 and different Rabs proteins were quantified. The graphs represent the proportion of HGF-555 in Rab4, Rab5, Rab7 and Rab11 compartment. ( d ) Lysates from cells stimulated with HGF for times indicated, pretreated for 20 min or not with Gö6976. The lysates were subjected to a GST-CRIB pull-down assay. The graph shows the fold increases over control 0 min. Data are presented as means±s.e.m. ( n =3, ** P <0.01 and NS: nonsignificant, Student’s t -test). ( e ) Lysates from cells transfected with control or PKCα siRNA and stimulated with HGF for the times indicated. The lysates were subjected to a GST-CRIB pull-down assay. The graph shows the fold increases over 0 min. Data are presented as means±s.e.m. ( n =3, * P <0.05 and NS: nonsignificant, Student’s t -test). ( f ) Lysates from cells transfected with control or Rab7 siRNA and stimulated with HGF for the times indicated. The lysates were subjected to a GST-CRIB pull-down assay. The graph shows the fold increases over Ct 0 min. Data are presented as means±s.e.m. ( n =3, ** P <0.01 and NS: nonsignificant, Student’s t -test). ( g ) Percentage of cells with Rac1 at the PM. Data are presented as means±s.e.m. ( n =5, ** P <0.01, Student’s t -test). Cells were transfected with a GFP-Rab7wt or GFP-Rab7NI, stimulated with HGF for 10 and 30 min, fixed and stained for Rac1. ( h ) Percentage of cells with ruffles. Data are presented as means±s.e.m. ( n =3, ** P <0.01, Student’s t -test). Cells were pretreated or not for 20 min with Gö6976 (Go) and stimulated with HGF as indicated, fixed and stained with cyanin3-phalloidin. Full size image It was shown previously in HeLa cells that c-Met traffics from a peripheral endosomal compartment to a perinuclear endomembrane compartment along the microtubule network and that this is facilitated by PKCα catalytic activity [14] . A similar process operated in MDA-468 cells since PKCα inhibition by Gö6976 or knockdown by siRNA, or microtubule stabilization by Taxol, did not prevent c-Met internalization but impaired its post-endocytic trafficking: at 30 min of HGF stimulation, HGF/c-Met vesicles appeared more dispersed in the cytoplasm and did not accumulate efficiently in the Rab7-positive PNE ( Fig. 2b,c and Supplementary Fig. 4a–c , Supplementary Movie 2 , right hand panel compared with the left hand panel). Thus, at 30 min in the presence of Gö6976, the proportion of c-Met colocalizing with GFP-Rab7 was reduced from 33 to 18%, and thus was restored to a level similar to that at 10 min (17%) indicating inhibition of endomembrane traffic ( Fig. 2c ). Consistent with this, at 30 min of HGF stimulation, c-Met colocalisation with Lamp1 was reduced from 36 to 15% in presence of Gö6976 ( Supplementary Fig. 4d ). Moreover, at 30 min in the presence of Gö6976, the extent of colocalization of each c-Met/Rab (4, 5, 7, 11) colocalization was restored to levels similar to that at 10 min ( Fig. 2c ). These results demonstrate that conditions impairing c-Met trafficking lead to c-Met retention at 30 min in the same compartments as seen at 10 min under control conditions, the PE ( Fig. 2c ). Moreover, the expression of the Rab7 dominant-negative GFP-Rab7N125I [44] , [45] ( Supplementary Fig. 4e ) or siRNA knockdown of Rab7 ( Supplementary Fig. 4f ) also impaired c-Met accumulation in the PNE ( Supplementary Fig. 4e,g ), consistent with the role of Rab7 in promoting RTK trafficking [5] . All together, these results indicate that these two compartments, the ‘PE’ with low Rab7 content and the ‘PNE’ with high Rab7 content, are distinct. Using these treatments, we then investigated whether modulating the post-endocytic trafficking of c-Met would have an influence on the Rac1 pathway. Interestingly, Gö6976, PKCα, Rab7 knockdown and Taxol had no effect at 0 or 10 min but significantly reduced Rac1 activation at 30 min in MDA-468 ( Fig. 2d–f , Supplementary Fig. 5a ). Consistent with this, Gö6976, PKCα knockdown ( Fig. 2h , Supplementary Fig. 5b,c ), the expression of GFP-Rab7N125I ( Fig. 2g ), Taxol ( Supplementary Fig. 5d ), and Rab7 knockdown ( Supplementary Fig. 5e ) had no effect at 0 or 10 min but led to a significant reduction in the percentage of cells with Rac1 at the cellular free edges and displaying membrane ruffles at 30 min. This reduction in the activation of Rac1 was not due to a reduction in c-Met activation since neither Gö6976, nor Taxol or Rab7 knockdown modified c-Met phosphorylation ( Supplementary Fig. 5f–h ). Importantly, we observed similar results in MDA-231, another invasive, basal-like human breast cell line. These cells displayed a similar long lasting wave of Rac1 activation upon HGF stimulation ( Supplementary Fig. 6a ). Moreover, the perturbation of c-Met trafficking to the Rab7-positive endosome, through inhibiting PKCα with Gö6976 ( Supplementary Fig. 6b ) or expressing Rab7N125I-GFP, had no effect at 0 or 10 min but led to a substantial reduction in the percentage of cells with Rac1 at the cellular free edges and inhibited Rac1 activation at 30 min ( Supplementary Fig 6c–e ). These results indicate that, although not absolutely required to trigger the Rac1 pathway, the trafficking of c-Met to the PNE is necessary to generate an optimal Rac1 activation, localization at the cellular free edges and an optimal formation of membrane ruffles. Rac1 activation is dependent on c-Met activity on the PNE Interestingly, we could visualize the c-Met-Rac1 pathway on PNEs. Thus, at 30 min of HGF stimulation, clear colocalization between perinuclear c-Met, Rac1 and Rab7 were observed in MDA-468 ( Fig. 3a ) and MDA-231 ( Supplementary Fig. 7 ). Consistent with this, colocalization between HGF-555 and Rac1-GFP were visualized in real-time imaging ( Supplementary Movie 3 ). 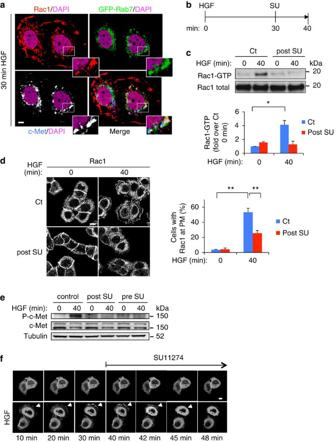Figure 3: c-Met activity on the PNE is required to sustain Rac1 signal in MDA-468 cells. (a) GFP-Rab7 (green) transfected cells were stimulated with HGF for 30 min and stained for Rac1 (red) and c-Met (white on bottom left picture, blue on merge picture). Colocalizations between Rac1, GFP-Rab7 and c-Met in vesicles appear in white in the merge picture. Scale bar, 10 μm. (b) Diagram showing protocol for (c–e). Cells were stimulated with HGF for 40 min and post treated or not with SU11274 (SU) 10 min before lysis or fixation. (c) The lysates were subjected to a GST-CRIB pull-down assay. The graph shows the fold increases over the 0 min control. Data are presented as means±s.e.m. (n=3, *P<0.05, Student’st-test). (d) Confocal sections of cells stained for Rac1. Scale bar, 10 μm. The graph shows the percentage of cells with Rac1 at the PM. Data are presented as means±s.e.m. (n=4, **P<0.01, Student’st-test). (e) Western blot for c-Met, phosphorylated c-Met (Y1234-35) and tubulin. (f) Confocal pictures extracted from theSupplementary Movie 5. Cells transfected with a GFP-actin plasmid were treated or not with HGF for 5 min and washed. The movies were acquired from 10 to 60 min. After 40 min, SU11274 was added. Images at indicated times are shown. The arrow indicates membrane ruffling. Scale bar, 10 μm. Figure 3: c-Met activity on the PNE is required to sustain Rac1 signal in MDA-468 cells. ( a ) GFP-Rab7 (green) transfected cells were stimulated with HGF for 30 min and stained for Rac1 (red) and c-Met (white on bottom left picture, blue on merge picture). Colocalizations between Rac1, GFP-Rab7 and c-Met in vesicles appear in white in the merge picture. Scale bar, 10 μm. ( b ) Diagram showing protocol for ( c – e ). Cells were stimulated with HGF for 40 min and post treated or not with SU11274 (SU) 10 min before lysis or fixation. ( c ) The lysates were subjected to a GST-CRIB pull-down assay. The graph shows the fold increases over the 0 min control. Data are presented as means±s.e.m. ( n =3, * P <0.05, Student’s t -test). ( d ) Confocal sections of cells stained for Rac1. Scale bar, 10 μm. The graph shows the percentage of cells with Rac1 at the PM. Data are presented as means±s.e.m. ( n =4, ** P <0.01, Student’s t -test). ( e ) Western blot for c-Met, phosphorylated c-Met (Y1234-35) and tubulin. ( f ) Confocal pictures extracted from the Supplementary Movie 5 . Cells transfected with a GFP-actin plasmid were treated or not with HGF for 5 min and washed. The movies were acquired from 10 to 60 min. After 40 min, SU11274 was added. Images at indicated times are shown. The arrow indicates membrane ruffling. Scale bar, 10 μm. Full size image This suggested that Rac1 is activated by c-Met on the PNE and further translocates to the PM to induce ruffle formation. c-Met was found to colocalize with p-c-Met (Y1234-35) staining on the PNE in MDA-468 cells, indicating that it remains activated in this compartment ( Supplementary Fig. 8 , top panel). To assess whether maintenance of c-Met activity on the PNE is necessary for HGF-dependent Rac1 activation and Rac1 localization at the cellular free edges, MDA-468 cells were treated with the c-Met inhibitor SU11274 once c-Met had reached the PNE. Thus, cells were stimulated with HGF for 30 min and incubation continued for further 10 min in the absence or presence of SU11274 ( Fig. 3b ); Strikingly, after this short time of treatment, Rac1 activation ( Fig. 3c ) as well as Rac1 localization at the PM ( Fig. 3d ) were reduced in the cells post treated with SU11274. Thus, Rac1 localization at the PM was detected in only 25% of the cells post treated with SU11274 as compared with over 50% of the non-treated cells ( Fig. 3d ). The efficiency of pre or post treatment by SU11274 was verified: SU11274 preincubation for 10 min and maintenance during the 40 min of HGF stimulation blocked c-Met phosphorylation; SU11274 post treatment (that is, added for the last 10 min of a 40-min HGF stimulation) also inhibited c-Met phosphorylation in the PNE ( Fig. 3e , Supplementary Fig. 8 , bottom panel). At 30 min of HGF treatment, internalized c-Met had trafficked to the PNE (see Figs 1d and 2a ) but remained accessible to the membrane permeable inhibitor SU11274. Although no obvious recycling of c-Met was observed by immunofluorescence in these cells, the possibility of reactivation at the PM of recycled c-Met was excluded by performing chase experiments where unbound HGF was washed away after 5 min of stimulation. Under these conditions, similar results were obtained as exemplified by Rac1 localization at the PM ( Supplementary Fig. 9a ). The influence of c-Met inhibition post endocytosis on actin dynamics at the leading edges of cells was analysed by live confocal imaging of MDA-468 cells transfected with GFP-actin. In parallel to the trafficking of HGF-555 containing vesicles towards the nucleus, it was observed that GFP-actin formed dynamic ruffles ( Supplementary Movie 4 ). Here again, reactivation of recycled c-Met at the PM was excluded since cells were stimulated with HGF-555 for 5 min to allow c-Met endocytosis and washed to remove unbound HGF before the start of the movie. Addition of SU11274 40 min post HGF led to a rapid loss of GFP-actin ruffling ( Supplementary Movie 5 , right hand panel, and Fig. 3f , bottom panel). In the absence of HGF, it was verified using GFP-actin that no ruffles formed ( Supplementary Movie 5 , left hand panel, and Fig. 3f , top panel). All together, these results demonstrate that HGF-dependent Rac1-sustained activation, Rac1 translocation to the cellular free edges and Rac1-dependent ruffling all require the retention of the c-Met perinuclear pool in an active state. They further show that Rac1 activation/translocation at the PM upon c-Met activation is a very dynamic process requiring sustained c-Met activity. We aimed to further demonstrate that c-Met recycling is not involved in Rac1 activation at 30 min of HGF stimulation. The rates of surface-biotinylated c-Met internalization and subsequent recycling were measured by streptavidin–agarose pulldown of surface-biotinylated c-Met as previously described [10] (see Methods). Briefly, MDA-468 cells were surface biotinylated on ice and were then stimulated with HGF at 37 °C for 7 or 30 min, followed by wash out of the medium and biotin cleavage at the cell surface. Cells were then reincubated in medium at 37 °C for 3 further minutes, followed or not followed by a second round of biotin cleavage at the cell surface, thus at 10 and 33 min. Streptavidin pulldown followed by c-Met western blot allowed the determination of the amount of the internalized biotinylated c-Met (one cleavage) and the amount of remaining internalized c-Met post-recycling (two cleavages). c-Met internalization was detected at 7 and 30 min of HGF stimulation ( Supplementary Fig. 9b ). At 10 min, the proportion of internalized c-Met was reduced with two cleavages compared with one cleavage, indicating a pool of c-Met had recycled back. However, no difference was seen at 30 min, indicating that c-Met is not recycling detectably at this time ( Supplementary Fig. 9b ). The levels of internalized c-Met were similar after one or two cleavages in the presence of the recycling inhibitor primaquine, confirming the recycling of c-Met at 10 min ( Supplementary Fig. 9b ). Interestingly, c-Met recycling at 10 min was impaired in cells treated with siRNA against Golgi-localized gamma ear-containing Arf-binding protein 3 (GGA3) ( Supplementary Fig. 9c ), consistent with the recently reported role of this molecule in promoting the recycling of a pool of internalized c-Met in HeLa cells post HGF stimulation [46] . While GGA3 knockdown had no effect on HGF-dependent Rac1 activation at 30 min, consistent with no c-Met recycling at this time, surprisingly, it led to a reduced Rac1 activation at 10 min HGF ( Supplementary Fig. 9d ). These results are consistent with a model where c-Met activation on the PNE is required to sustain Rac1 activation at 30 min of HGF stimulation without the need of c-Met recycling. They further suggest that GGA3-dependent c-Met recycling plays a role in Rac1 activation at 10 min of HGF stimulation. As internalization and recycling are required at 10 min, our results suggest that a dynamic turnover between the PE and the PM are required to efficiently trigger the early wave of Rac1 activation. All together, these results indicate further that mechanisms regulating c-Met-Rac1 pathway are very different in the PNE versus PE. c-Met traffic correlates with HGF-dependent cell migration We then assessed the influence of PKCα inhibition on HGF-dependent MDA-468 cell migration, using Gö6976 or PKCα siRNA knockdown. Both treatments significantly reduced HGF-dependent MDA-468 cell transwell migration ( Fig. 4a,b ). The maintenance of c-Met activation during the time of this assay was verified ( Supplementary Fig. 10a ). Moreover, Rab7 siRNA knockdown also impaired HGF-dependent cell transwell migration ( Supplementary Fig. 10b ). However, GGA3 siRNA knockdown did not reduce cell migration to the same extent ( Supplementary Fig. 10c ). These results suggested that the trafficking of c-Met to the PNE is required for HGF-dependent cell migration. 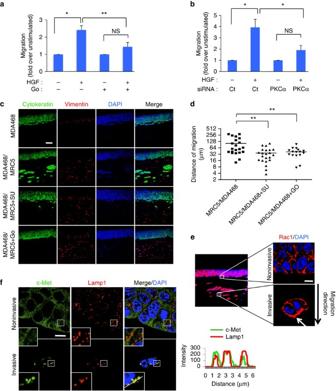Figure 4: c-Met trafficking correlates with HGF-dependent MDA-468 cell migration. (a) Migration across transwells of cells stimulated or not with HGF, pretreated or not with Gö6976 (Go). The graph shows the fold increases over unstimulated cells. Data are presented as means±s.e.m. (n=3, *P<0.05, **P<0.01 and NS: nonsignificant, Student’st-test). (b) Migration across transwells of cells transfected with control or siPKCα siRNA and stimulated or not with HGF. The graph shows the fold increases over unstimulated cells. Data are presented as means±s.e.m. (n=3, *P<0.05 and NS: nonsignificant, Student’st-test). (c) Cells were grown in organotypic cultures for 14 days under the conditions indicated, fixed, included in paraffin, sectioned (8 μm) and stained for cytokeratin (green), vimentin (red) and DAPI (blue). A representative confocal section is shown. Scale bar, 100 μm. (d) Quantification of cell invasion in the extracellular matrix of organotypic cultures. Squares or triangles are the means of the distance of migration of the five most migratory colonies in the gel/microscopic field. Twenty-three fields per condition were counted (**P<0.01, one-way analysis of variance test). (e) Confocal sections of organotypic cultures of MDA-468 cells in presence of MRC5 fibroblasts at 14 days of culture, and stained for Rac1 (red) and DAPI (blue) (right panel). The top right picture shows MDA-468 cells at the interface of the epithelial layer and the gel (noninvasive). The bottom right picture shows MDA-468 cells inside the gel (invasive). The arrow indicates Rac1 at the cell leading edge. Scale bar, 10 μm. (f) Confocal sections of organotypic cultures of MDA-468 cells in presence of MRC5 fibroblasts at 14 days of culture, and stained for c-Met (green), Lamp1 (red) and DAPI (blue). The top pictures show MDA-468 cells at the interface of the epithelial layer and the gel (noninvasive). The bottom right picture shows MDA-468 cells inside the gel (invasive). Scale bar, 10 μm. Colocalizations appear in yellow. Plots of the intensity profiles, at different emission wavelengths corresponding to the signals of c-Met and Lamp1 in an invasive cells, of a set of pixels distributed on a line drawn across vesicles (shown in the magnification) are shown. Figure 4: c-Met trafficking correlates with HGF-dependent MDA-468 cell migration. ( a ) Migration across transwells of cells stimulated or not with HGF, pretreated or not with Gö6976 (Go). The graph shows the fold increases over unstimulated cells. Data are presented as means±s.e.m. ( n =3, * P <0.05, ** P <0.01 and NS: nonsignificant, Student’s t -test). ( b ) Migration across transwells of cells transfected with control or siPKCα siRNA and stimulated or not with HGF. The graph shows the fold increases over unstimulated cells. Data are presented as means±s.e.m. ( n =3, * P <0.05 and NS: nonsignificant, Student’s t -test). ( c ) Cells were grown in organotypic cultures for 14 days under the conditions indicated, fixed, included in paraffin, sectioned (8 μm) and stained for cytokeratin (green), vimentin (red) and DAPI (blue). A representative confocal section is shown. Scale bar, 100 μm. ( d ) Quantification of cell invasion in the extracellular matrix of organotypic cultures. Squares or triangles are the means of the distance of migration of the five most migratory colonies in the gel/microscopic field. Twenty-three fields per condition were counted (** P <0.01, one-way analysis of variance test). ( e ) Confocal sections of organotypic cultures of MDA-468 cells in presence of MRC5 fibroblasts at 14 days of culture, and stained for Rac1 (red) and DAPI (blue) (right panel). The top right picture shows MDA-468 cells at the interface of the epithelial layer and the gel (noninvasive). The bottom right picture shows MDA-468 cells inside the gel (invasive). The arrow indicates Rac1 at the cell leading edge. Scale bar, 10 μm. ( f ) Confocal sections of organotypic cultures of MDA-468 cells in presence of MRC5 fibroblasts at 14 days of culture, and stained for c-Met (green), Lamp1 (red) and DAPI (blue). The top pictures show MDA-468 cells at the interface of the epithelial layer and the gel (noninvasive). The bottom right picture shows MDA-468 cells inside the gel (invasive). Scale bar, 10 μm. Colocalizations appear in yellow. Plots of the intensity profiles, at different emission wavelengths corresponding to the signals of c-Met and Lamp1 in an invasive cells, of a set of pixels distributed on a line drawn across vesicles (shown in the magnification) are shown. Full size image In order to better approach physiological conditions, we further analysed MDA-468 cell motility in three-dimensional organotypic cultures, which allow cancer cell invasion into a reconstituted extracellular matrix embedded with fibroblasts [47] . The fibroblasts chosen for the experiments are the cell line MRC5, as they secrete HGF [48] . Indeed, conditioned medium from MRC5 cells was able to stimulate c-Met phosphorylation in MDA-468 cells, which was prevented by incubation with SU11274 ( Supplementary Fig. 10d ). It also stimulated c-Met endocytosis ( Supplementary Fig. 10e ) and Rac1 localization at the cellular free edges ( Supplementary Fig. 10f ). MDA-468 breast cancer cells were applied to the top of gels and cultures were maintained for 14 days (see diagram Supplementary Fig. 10g ). Paraffin-embedded sections were then immunostained for cytokeratin and vimentin to clearly distinguish between cancer cells and MRC5 cells, respectively ( Fig. 4c ). In the absence of MRC5 cells, MDA-468 cells did not invade the matrix, while in the presence of MRC5, MDA-468 cells invaded the gel with an average distance of migration of 103 μm over this 14-day period. Incubation of MDA-468 cells in SU11274 reduced the distance of migration to an average of 36 μm ( Fig. 4d ), indicating that c-Met activity is required for efficient cell invasion. Interestingly, incubation of MDA-468 cells in Gö6976 reduced the invasion of MDA-468 cells to the same extent (41 μm) ( Fig. 4c,d ), indicating that PKCα activity, and thus possibly intracellular c-Met trafficking, is required. Interestingly, Rac1 localized at the leading edge of invasive cells only ( Fig. 4e ). Strikingly, c-Met staining appeared accumulated in large punctate structures in invasive cells. Moreover, a significant proportion of c-Met vesicles colocalized with Lamp1 in the perinuclear area ( Fig. 4f ), consistent with the idea that the trafficking to the PNE may be important for cell motility. All together, these results suggest that PKCα-dependent c-Met trafficking to the PNE is required for HGF-dependent MDA-468 cell motility. Rac1-sustained activation depends on Vav2 and PI3K activity We sought to determine why c-Met needs to localize to the perinuclear compartment to trigger an optimal stimulation of the Rac1 pathway and subsequent cell motility. As it is not due to a different strength in c-Met activation/tyrosine phosphorylation (see Supplementary Fig. 5f–h ), we hypothesized that c-Met may have differential access to Rac1 upstream effectors in the perinuclear and the peripheral compartments. We asked whether Rac1 activation by c-Met could be mediated through a specific GEF in the PNE. We first investigated Tiam1, previously reported to control HGF/c-Met-dependent Rac1 activation and membrane ruffles [9] . However, upon Tiam1 knockdown, no difference in Rac1 activation was detected at 10 or 30 min of HGF stimulation in this breast cancer cell model ( Supplementary Fig. 11a,b ). We then investigated Vav2, which represented a potential candidate as it had been shown to regulate a late phase of EGF-dependent RhoB stimulation [49] . Strikingly, in Vav2 knocked-down cells, Rac1 activation was blocked at 30 min but not at 10 min of HGF stimulation ( Fig. 5a ). Consistent with this, colocalization was observed between c-Met and Vav2 in the perinuclear location at 30 min of HGF stimulation ( Fig. 5b ). Real-time confocal imaging showed that the initially diffuse GFP-Vav2 signal became progressively punctate upon time of HGF-555 stimulation ( Supplementary Movie 6 ). These punctate structures in fact corresponded to vesicles where GFP-Vav2 colocalized with HGF-555. This colocalization increased over time such that all HGF-555-positive perinuclear vesicles colocalized with Vav2-GFP ( Supplementary Movie 6 ), indicating an optimal recruitment of Vav2 with c-Met while located on the PNE. Finally, knocking down Vav2 reduced HGF-stimulated cell migration significantly ( Fig. 5c ). Since it had been reported that Vav2 expression affects EGFR endocytosis and degradation [50] , we assessed this for c-Met and found that c-Met degradation ( Supplementary Fig. 11c ) and endocytosis ( Supplementary Fig. 11d ) were not affected. Importantly, we observed similar results in MDA-231 where Vav2 knockdown inhibited Rac1 activation at 30 min of HGF stimulation while it had no effect at 10 min ( Supplementary Fig. 11e ). 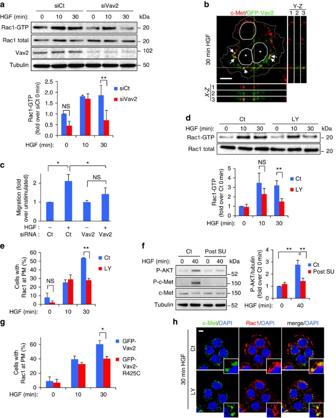Figure 5: Rac1-sustained activation depends on Vav2 and PI3K activity in MDA-468 cells. (a) Cells, transfected with control or Vav2 siRNAs, were stimulated with HGF for the indicated times, followed by GST-CRIB pull-down. Fold increases over unstimulated cells are shown Data are presented as means±s.e.m. (n=3, **P<0.01 and NS: nonsignificant, Student’st-test). (b) GFP-Vav2 (green) transfected cell were stimulated with HGF for 30 min and stained for c-Met (red). Orthogonal reconstructions of serial confocal slices are shown (y-zandx-zaxis with 1: c-Met, 2: Vav2, 3: merge of 1 and 2) alongside one z-slice taken in the middle of the cells. The perpendicular yellow lines on the section indicate from where the orthogonal views where built. Colocalizations between GFP-Vav2 and c-Met in vesicles appear in yellow. The white circles represent the nuclei. * transfected cells. Scale bar, 10 μm. (c) Migration across transwells of cells transfected with control or Vav2 siRNA and stimulated or not with HGF. Fold increases over siControl, no HGF are shown. Data are presented as means±s.e.m. (n=5, *P<0.05, Student’st-test). (d) Cells pretreated or not with LY294002 (LY) for 10 min, were stimulated with HGF for the times indicated. The lysates were subjected to GST-CRIB pull-down. Fold increases over control 0 min at each time of HGF stimulation are shown. Data are presented as means±s.e.m. (n=3, **P<0.01, Student’st-test). (e) Percentage of cells with Rac1 at the PM. Data are presented as means±s.e.m. (n=4, **P<0.01, Student’st-test). Cells, pretreated or not with LY294002 (LY) for 10 min, were stimulated with HGF for the times indicated, fixed and stained for Rac1. (f) Cells were stimulated with HGF for 40 min and post treated or not with SU11274 (SU) 10 min before lysis (seeFig. 3bfor protocol). Western blot for P-AKT, P-c-Met (Y1234-35), c-Met and tubulin were performed. Fold increases over control, no HGF are shown. Data are presented as means±s.e.m. (n=3, **P<0.01, Student’st-test). (g) Percentage of cells with Rac1 at the PM. Data are presented as means±s.e.m. (n=3, *P<0.05, Student’st-test). Cells were transfected with GFP-Vav2wt or GFP-Vav2-R425C, stimulated with HGF for 10 and 30 min, fixed and stained for Rac1. (h) Confocal sections of cells stimulated with HGF for 30 min, pretreated for 10 min or not with LY294002 (LY) and stained for c-Met (green), Rac1 (red) and DAPI (blue). Scale bar, 10 μm. Figure 5: Rac1-sustained activation depends on Vav2 and PI3K activity in MDA-468 cells. ( a ) Cells, transfected with control or Vav2 siRNAs, were stimulated with HGF for the indicated times, followed by GST-CRIB pull-down. Fold increases over unstimulated cells are shown Data are presented as means±s.e.m. ( n =3, ** P <0.01 and NS: nonsignificant, Student’s t -test). ( b ) GFP-Vav2 (green) transfected cell were stimulated with HGF for 30 min and stained for c-Met (red). Orthogonal reconstructions of serial confocal slices are shown ( y - z and x - z axis with 1: c-Met, 2: Vav2, 3: merge of 1 and 2) alongside one z-slice taken in the middle of the cells. The perpendicular yellow lines on the section indicate from where the orthogonal views where built. Colocalizations between GFP-Vav2 and c-Met in vesicles appear in yellow. The white circles represent the nuclei. * transfected cells. Scale bar, 10 μm. ( c ) Migration across transwells of cells transfected with control or Vav2 siRNA and stimulated or not with HGF. Fold increases over siControl, no HGF are shown. Data are presented as means±s.e.m. ( n =5, * P <0.05, Student’s t -test). ( d ) Cells pretreated or not with LY294002 (LY) for 10 min, were stimulated with HGF for the times indicated. The lysates were subjected to GST-CRIB pull-down. Fold increases over control 0 min at each time of HGF stimulation are shown. Data are presented as means±s.e.m. ( n =3, ** P <0.01, Student’s t -test). ( e ) Percentage of cells with Rac1 at the PM. Data are presented as means±s.e.m. ( n =4, ** P <0.01, Student’s t -test). Cells, pretreated or not with LY294002 (LY) for 10 min, were stimulated with HGF for the times indicated, fixed and stained for Rac1. ( f ) Cells were stimulated with HGF for 40 min and post treated or not with SU11274 (SU) 10 min before lysis (see Fig. 3b for protocol). Western blot for P-AKT, P-c-Met (Y1234-35), c-Met and tubulin were performed. Fold increases over control, no HGF are shown. Data are presented as means±s.e.m. ( n =3, ** P <0.01, Student’s t -test). ( g ) Percentage of cells with Rac1 at the PM. Data are presented as means±s.e.m. ( n =3, * P <0.05, Student’s t -test). Cells were transfected with GFP-Vav2wt or GFP-Vav2-R425C, stimulated with HGF for 10 and 30 min, fixed and stained for Rac1. ( h ) Confocal sections of cells stimulated with HGF for 30 min, pretreated for 10 min or not with LY294002 (LY) and stained for c-Met (green), Rac1 (red) and DAPI (blue). Scale bar, 10 μm. Full size image Thus, we identified Vav2 as a specific GEF for the c-Met-Rac1 pathway in the PNE. Moreover, the late phase Rac1 activation driven through c-Met specifically via Vav2 from the PNE is a necessary element of HGF-induced migration. The PI3K pathway is a major c-Met effector and a regulator of Rac-GEF activities [51] . As Vav2 has a PH domain, and is potentially regulated by the binding to the PI3K product phosphatidylinositol 3,4,5-trisphosphate (PIP3), we investigated the PI3K pathway. Interestingly, pretreatment of cells with the PI3K inhibitor LY294002 had no effect on the basal (0 min) or on the HGF-dependent Rac1 activation and Rac1 translocation at the cellular free edges at 10 min, but it did lead to a significant reduction at 30 min ( Fig. 5d,e ). An acute post treatment with SU11274 at 30 min of HGF stimulation led to a significant reduction in phosphorylation of the PI3K downstream effector AKT (from 2.8-fold to 1.4-fold) ( Fig. 5f ). It was verified that LY294002 did not prevent c-Met internalization or accumulation in the PNE at 30 min of HGF stimulation, consistent with the hypothesis that PI3K plays a role in c-Met-Rac1 pathway directly on the PNE rather than through influencing c-Met trafficking. Moreover, in confocal live imaging, we detected colocalization between the phosphatidylinositol 3-kinase regulatory subunit alpha (P85α-GFP) and HGF-555 in PNEs ( Supplementary Movie 7 ). To assess the requirement of PI3K for the correct input of Vav2 in c-Met-dependent Rac1 activation at 30 min of HGF stimulation, we used the mutant GFP-Vav2-R425C carrying a point mutation in the PH domain compromising binding to PIP3. Following 30 min of HGF treatment in GFP-Vav2-R425C-expressing MDA-468 cells, the percentage of cells with Rac1 at the cellular free edges was significantly reduced to 40% compared with 60% in Vav2-GFP expressing cells; no such effect was observed at 0 and 10 min of HGF treatment ( Fig. 5g ). This result indicates that the Vav2 PH domain is required for the optimal c-Met-Rac1 pathway in the PNE and suggests that HGF regulates Vav2 activity through PI3K activation. Finally, although LY294002 prevented Rac1 activation ( Fig. 5d ) and translocation to the cellular free edges at 30 min of HGF stimulation ( Fig. 5e ), it did not prevent the colocalization between c-Met and Rac1 in the PNE ( Fig. 5h ), thus suggesting further that PI3K input is to activate colocalized Rac1. These results indicate that c-Met requires PI3K activity to activate Rac1 through Vav2 only when signalling from the PNE and suggest that c-Met can activate PI3K on the PNE, which leads to Vav2-dependent Rac1 activation, and translocation to the cellular free edges, leading to membrane ruffles formation. Upon HGF stimulation, in MDA-468 basal-like breast cancer cells, endocytosis is required for the stimulation of Rac1, subsequent actin reorganization at the leading edge and directed cell migration, consistent with previous findings [9] , [10] . Our results indicate that, in these cells, c-Met triggers the activation of Rac1 from both peripheral and perinuclear endomembranes (PE/PNE). However, c-Met needs to traffic to the PNE to sustain Rac1 activity and trigger optimal membrane ruffling. The process is very dynamic since acute inhibition of c-Met, when it is localized on the PNE, leads to a rapid reduction of Rac1 localization at the cellular free edges and membrane ruffling loss. Although endosomal signalling of receptors has become increasingly recognized [1] , [2] , [3] , [4] , [5] , [6] , underlying principles are poorly understood. One paradigm concerns access to specific effectors as evidenced by the p14–MP1 complex [7] , which assembles MEK1 and ERK1/2 on late endosomes, the Rab5 effector Appl1, which recruits AKT and its substrate GSK-3β on ‘Appl endosomes’ [8] and the FYVE domain protein SARA, which recruits TGFβ receptor to the endosome [52] , [53] . Endosomes can also provide protection against negative regulators, such as phosphatases [54] , as shown for the c-Met-STAT3 pathway [16] . The prevailing view is that endosomes concentrate signalling molecules in defined intracellular regions and, as a consequence, specific signals are generated or sustained. Although some studies have reported endosome-specific signalling, such as AKT-GSK-3β pathway on Appl1 endosomes [8] , MEK1-ERK1/2 in the late endosome [7] , signalling from endosomes generally has been distinguished from signalling from the PM. For example, ERK1/2 signalling may require different scaffolds at the PM (KSR and IQGAP1) [55] than on endosomes (MP1-p14 complex) [7] . Notably, we have extended the concept of compartmentally resolved signals by identifying a growth factor receptor triggering the same signal output, from distinct endomembrane compartments via different effectors’ mechanisms. Indeed PI3K activity and the expression of the GEF Vav2 are required for the optimal stimulation of Rac1 by c-Met when localized in the PNE but not in the PE. Thus, there is a requirement for c-Met post early endosomal trafficking to sustain the Rac1 promigratory pathway, reflecting the engagement of the specific effectors PI3K and Vav2 (see Supplementary Fig. 11f ). The visualization of Vav2 and p85-PI3K on the HGF-555 (as a marker of the ligand bound c-Met)-positive PNE is consistent with this model. We propose that HGF-bound c-Met traffics to the PNE (under the control of PKCα activity but not of PI3K activity or Vav2 expression) where it can activate PI3K and associate with Vav2. The mechanisms involved in Vav2 activity are poorly understood. On the one hand, the phosphorylation of highly conserved tyrosine residues in the acidic domain of Vav2 has been shown to positively regulate Vav2 GDP/GTP exchange activity [56] , [57] , [58] . On the other hand, a Vav2-intact PH domain [59] , [60] was reported required for Vav2 activity. In our model, Vav2 is activated after binding to the locally produced PIP3, as evidenced by the inability of the PH domain mutant to sustain the signal, and it is then able to activate Rac1 locally, followed by a rapid translocation of active Rac1 to the cellular free edges triggering membrane ruffling. Finally, Vav2 has been reported to be required for the local activation of PI3K at cellular protrusions [60] , suggesting that in our model, Vav2 may exert a positive feedback on PI3K activation, thus amplifying c-Met-dependent Rac1 activation in the PNE. It was previously shown that, although endocytosis alone is sufficient to support ERK1/2 nuclear accumulation upon HGF stimulation, STAT3 nuclear accumulation requires further microtubule traffic of c-Met to a PNE [16] . Here, it is not the access to specific effectors in a particular endosome that controls STAT3 nuclear accumulation; rather, it is the juxtanuclear activation of a weak signal that allows the required threshold of phosphorylation for nuclear entry. c-Met is able to activate STAT3 from different compartments including the PM but the signal is too weak to trigger its access to the nucleus through diffusion in a phosphatase-rich environment. c-Met trafficking to the perinuclear area allows local phosphorylation of STAT3, which is then above the threshold required to enable nuclear entry. By contrast, for Rac1, different activation mechanisms are engaged depending on the c-Met location in PE and PNE; different effectors are accessing the activated receptor in these compartments. Thus, c-Met trafficking to the PNE regulates two major signal outputs, STAT3 and Rac1, but the mechanisms involved are distinct. In addition, it was shown previously that, unlike STAT3, ERK1/2 nuclear accumulation requires c-Met trafficking to the PE but not to the PNE [16] . Therefore, for one given receptor, there can be a variety of mechanisms exploiting its trafficking to control signal output. It is evident then that the controls exerted on receptor traffic itself will influence the nature of signals emanating from the receptor. Endosomal signalling has emerged as playing a major role in the control of specific cell functions, such as cell migration [9] , [15] , [16] , [17] . Our results suggest that not only c-Met endocytosis but also further trafficking to a PNE plays a role in cell motility. Inhibition of PKCα, which normally promotes c-Met post-endocytic trafficking, inhibited cell migration in three-dimensional organotypic cultures. Traffic of c-Met has been shown to be important in migratory behaviour in conventional cell culture systems [15] , [16] . Here we have shown that this is in part linked to a Rac1 pathway that is triggered by active HGF-c-Met complexes localized to specific intracellular compartments from where they stimulate specific effectors. Importantly, our results suggest that the trafficking requirements of c-Met in invasive behaviour are retained. In addition to operating as signalling platforms, endosomes may contribute to the promotion of an intrinsic polarity of the migrating cells, at the front, as evidenced by RTK signalling in Drosophila border cells [17] , or at the rear, as seen for endo180-Rho-Rock-MLC2 signalling [61] . This spatial restriction of RTK signalling may operate via PM–endosome trafficking cycles. Thus, in addition to endocytic regulators such as clathrin, dynamin or cbl [9] , [15] , [16] , [17] , recycling regulators such as Rab11 or Rab-coupling proteins have been implicated in cell migration through promoting the recycling of Drosophila RTK [17] or EGFR [62] , respectively. Oncogenic, constitutively active c-Met forms, mutated in the kinase domain (M1268T or D1246N) [63] , [64] , [65] , [66] , undergo such shuttling, leading to persistent endosomal Rac1 signalling, actin reorganization, enhanced cell migration and metastasis [10] . c-Met wild type has mostly been described to get progressively degraded upon HGF stimulation [14] . However, the recycling of a proportion of internalized c-Met, under the control of Rab-coupling protein in various cells expressing mutant p53 (ref. 67) [67] , or under the control of GGA3 in HeLa cells [46] , has been reported. Interestingly, we also have detected that, in MDA-468 cells following 10 min of stimulation, 40% of c-Met recycles, under the control of GGA3. Moreover, GGA3 siRNA knockdown lead to a reduction of Rac1 activation upon 10 min of HGF stimulation, indicating that c-Met recycling is in fact required for the early phase of Rac1 activation. Thus, at 10 min, c-Met internalization and recycling appear required suggesting that, at this early time of stimulation, a shuttling PE PM is required to stimulate Rac1 acutely. As c-Met has been found to recycle into dorsal ruffles at an early phase of HGF stimulation in MDCK cells [13] , one possibility is that this early shuttling operates between PE and dorsal ruffles in MDA-468 cells. Nevertheless, this early phase of acute c-Met-Rac1 pathway appears insufficient to trigger cell migration as GGA3 siRNA knockdown is not able to fully reduce HGF-dependent cell transwell migration of MDA-468 cells. Importantly, no recycling was detected at 30 min. This result is consistent with our model that c-Met needs to traffic to the PNE to trigger an optimal Rac1 activation and subsequent cell motility. Interestingly, however, the perinuclear c-Met endosomes appear polarized on the side of the nucleus facing the cells’ free edges. Thus, c-Met stimulation of Rac1 pathway from the PNE may maintain a spatial organization of the signalling complexes towards the leading edge, triggering a local modification of the actin cytoskeleton and formation of lamellipodia. In conclusion, we describe here a novel endosomal signalling mechanism whereby one signal output, Rac1, is stimulated through distinct pathways by the same RTK depending on which endosome it is localized to in the cell. One of these endosomal-specific pathways involving PI3Kinase and Vav2 is necessary to sustain the signalling output leading to optimal cytoskeleton modelling and breast cancer cell migration. Interestingly, the role of Rho GEFS in cancer is emerging, including Vav2 (ref. 68) [68] . Moreover, Vav2 recently was shown to be required for lung-specific metastasis of breast cancer [69] . As broad inhibition of c-Met by specific tyrosine kinase inhibitors may lead to tumour resistance, such as is seen in the clinic with other RTK inhibitors, targeting localized effectors, such as Vav2 in c-Met-driven invasive breast tumours, may represent alternative therapeutic solutions. Cell culture, transfection, RNA interference MDA-468 cells and MDA-231 cells (ATCC) were cultured in DMEM (Sigma) supplemented with 10% fetal bovine serum and L-glutamine (2mM) and maintained at 37 °C in a humidified 8% CO 2 atmosphere. Transfections were performed using Amaxa technology (kit V, Lonza). Two different RNA interferences (RNAis) were used for: Rac1 knockdown (Dharmacon, Inc.): Rac1-1: 5′-UAAGGAGAUUGGUGCUGUA-3′; Rac1-2: 5′-CGGCACCACUGUCCCAACA-3′. Rab7 knockdown (Dharmacon, Inc.): Rab7A-1: 5′-CUAGAUAGCUGGAGAGAUG-3′; Rab7A-3: 5′-AAACGGAGGUGGAGCUGUA-3′. The more efficient RNAi of a pool of four oligos was used for Tiam1 (5′-GAACCGAAGCUGUAAAGAA)-3′, Vav2 (5′-AUCCAAAUCUCCCGUUAUA-3′) and GGA3 (5′-GAGGAGAAGUCCAAGCUUU-3′) (Dharmacon, Inc.). One clathrin heavy chain siRNA was used (Qiagen): 5′-AAGAAGGCTCGAGAGTCCTAT-3′. One previously described PKCα siRNA was used [15] . The sequence of the control RNAi does not match to any known sequence (Qiagen). For all experiments, 1 μg of RNAi was used. The plasmid GFP-actin was obtained from Dr Maddy Parsons, Kings College, London. The plasmids GFP-Vav2 and GFP-Vav2-R425C were obtained from László Buday, Semmelweis University, Budapest. The plasmid YFP-CRIB-CFP was obtained from Giorgio Scita, IFOM-IEO Campus, Milan. The plasmid p85a-GFP was obtained from Bart Vanhaesebroeck, Barts Cancer Institute, Queen Mary University, London. The plasmid GFP-Rab7 and GFP-Rab7NI were obtained from Miguel Seabra, Imperial College, London. The plasmids GFP-Rab4, GFP-Rab5, GFP-Rab11 were as described previously [70] . Reagents Purified human recombinant HGF (100 ng ml −1 ) was obtained from R&D Systems. SU11274 (2 μM), Gö6976 (1 μM), Taxol (5 μM) and LY294002 (10 μM) were obtained from Calbiochem, dynasore (80 μM) from Sigma and cyanin 3-conjugated phalloidin from Molecular Probes. The following primary antibodies ( Supplementary Table 1 ) were used: goat polyclonal anti-c-Met (R&D Systems) and anti-Rab7 (Santa Cruz); mouse monoclonals anti-c-Met (Novocastra), anti-Rac1 (Cytoskeleton and Upstate Biotechnology), -PKCα and -GGA3 (BD Transduction Laboratories), -tubulin (Sigma), -vimentin (Dako), -p85 subunit of phosphoinositide-3 kinase (PI3K) (P13020, Transduction Laboratories); rabbit polyclonals anti-EEA1 (Santa Cruz), -phospho-c-Met (Tyr 1234-1235) (Cell signaling), -phospho-c-Met (Tyr 1234-1235) (clone 421, in house LRI CR-UK), -phospho-c-Met (Tyr 1349) (Cell signaling), -Lamp1 (Abcam), -Tiam1 (Invitrogen), -Vav2 (Santa Cruz), -pan-cytokeratin (Dako), -phospho-AKT(ser473) (Cell signaling). The following secondary antibodies were used: for immunofluorescence: Alexa-488 labelled anti-goat, anti-rabbit or anti-mouse IgG (1/500, Molecular Probes), and Cy3-coupled anti-goat, anti-rabbit or anti-mouse IgG and Cy5-coupled anti-rabbit IgG (1/500, Jackson Immunoresearch); for western blot: both anti-mouse and anti-rabbit IgG secondary antibodies were coupled to horseradish peroxidase, purchased from Amersham and used at a dilution of 1/1,000. Immunofluorescence and confocal microscopy analyses Cells were plated in 24-well plates (5 × 10 4 per well) onto glass coverslips and stimulated the following day in full medium as indicated. Cells were starved 24 h prior to dynasore incubation. Dynasore was added 30 min prior to HGF and other inhibitors 10 min prior to HGF. Immunofluorescence was performed as described previously [16] . For Lamp1 staining, cells were permeabilized in Tris buffer saline (TBS) containing 0.2% Tween 20 for 20 min, blocked for 15 min in TBS containing 0.2% Tween, 1% BSA, 10% FCS, 0.3 M glycine. Lamp1 and secondary antibodies were then incubated in TBS containing 0.2% Tween. Confocal microscopy was performed as described [16] using a confocal laser-scanning microscope (LSM510 or LSM710, Carl Zeiss Inc.). Each image corresponds to a single section of 0.8 μM thickness. Orthogonal views from Z-stack have been organized in the ImageJ software (National Institute of Health, USA). For image quantitations, picture fields were chosen arbitrarily based on DAPI (4,6-diamidino-2-phenylindole) staining only. The counting of cells with Rac1 at the PM or with ruffles, were performed on at least 100 cells in each experiment. The percentages of colocalizations were determined using the Zen software (Carl Zeiss Inc.) on unsaturated images. Live cell confocal imaging was performed on LSM510 or LSM710 confocal microscopes equipped with a 63 × 1.4 Plan-Apochromat oil immersion objective and an incubation chamber for temperature and CO 2 control. Briefly, 2 days after transfection, cells were stimulated with HGF or Alexa Fluor® 555-conjugated HGF (HGF-555) [16] for 5 min. Cells were washed three times in phenol red-free DMEM supplemented with 10% of fetal bovine serum and acquisition of the movie started after 5 min (thus 10 min after HGF). Cells were treated or not with SU11274, 40 min after HGF treatment. Acquisition of the pictures was taken every 14 s with a section depth of 1.1 μM. Western blots and densitometry analysis Cells were harvested in radioimmunoprecipitation buffer (RIPA) or directly in Laemmli sample buffer (Invitrogen) and boiled for 10 min. Samples were loaded on 4–12% gradient polyacrylamide gels (Invitrogen). Separated proteins were transferred to a 0.45-μm nitrocellulose transfer membrane (Whatman). Protein loading was checked by staining with Ponceau Red. Membranes were then blotted with appropriate first antibodies at a dilution of 1:1,000. Specific binding of antibodies was detected with appropriate peroxidase-conjugated secondary antibodies and visualized by enhanced chemiluminescence detection (GE Healthcare). Densitometric analyses of immunoblots were performed using ImageJ 1.47v (National Institute of Health). Full blots are included in the supplementary information ( Supplementary Fig. 12–15 ). Rac1 activation assay The levels of Rac1-GTP were measured by precipitation using the GST-CRIB domain of PAK1 with the Rac1 Activation Assay Biochem Kit (Cytoskeleton), according to the manufacturer’s instructions. Bound GTP-Rac1 was detected by western blot with an anti-Rac1 antibody. Recycling assay On ice, cell surface proteins were labelled with 0.2 mg ml −1 sulpho-NHS-SS-biotin (sulpho-NHS)-SS-biotin; Pierce) in PBS for 45 min. Labelled cells were washed with cold PBS and incubated at 37 °C with HGF in culture medium, to allow protein trafficking. At 7 or 30 min, the medium was aspirated and the dishes were transferred to ice and washed with cold PBS. Biotin was removed from proteins remaining at the cell surface by reduction for 15 min with 180 mM of the membrane-impermeant reducing agent MesNa (sodium 2 mercaptoethane sulphonate, Sigma) in 50 mM Tris and 100 mM NaCl at pH 8.6. MesNa was quenched by the addition of 180 mM iodoacetamide (IAA, Sigma) for 10 min. To measure the proportion of the internalized Met that recycles back to the cell surface, the internalized fraction was chased from the cells treated with HGF during 7 min (time point 7+3 min on figure) or 30 min (time point 30+3 min on figure) by returning them to 37 °C for 3 min. Cells were then returned to ice and biotin was removed from recycled proteins by a second reduction with MesNa. Unreacted MesNa was quenched with IAA and cells were lysed. Lysates were passed three times through a 27-gauge needle and clarified by centrifugation (17,000 g ); equal protein amounts (100 μg) received streptavidin–agarose beads (upstate) and were agitated at 4 °C for 2 h; beads were collected by centrifugation (7,000 g ), washed in lysis buffer and proteins were extracted by heating at 95 °C with sample buffer. In each recycling assay, two controls were carried out. To measure the total c-Met at the surface (TS), biotinylated cells at 4 °C were lysed without biotin reduction. To verify the efficiency of the surface biotin removal, the biotin reduction and MesNa quenching steps were carried out on cells that had remained on ice (time 0) and lysis was carried out. Equivalent volumes were analysed in a c-Met western blotting assay and densitometric analyses were carried out. Percent recycled c-Met was determined by quantifying IB and subtracting the amount recovered from a similarly processed sample that did not undergo a second round of reduction (representing total pool of internalized Met) divided by the total pool of internalized Met. Transwell migration assay Twenty-four hours before the assay, cells were serum deprived. The transwell (8 μM pore size, Corning) underside was coated with 70 μl fibronectin (1:100 in PBS, Sigma) for 30 min and dried. A quantity of 2 × 10 4 cells were added to the upper well with medium containing 1% serum, supplemented with 0.1% BSA, with drug or DMSO. The lower well contained 600 μl of cell culture medium containing 1% serum with drug or DMSO or HGF. After 4 h of culture (37 °C, 8% CO 2 ), cells remaining in the upper well were removed using a cotton bud. The inserts were fixed in 4% paraformaldehyde and stained with haematoxylin for 5 min. Cells that had migrated on the membrane underside were counted in 10 random fields ( × 20 objective, Zeiss Axiophot microscope). Organotypic cultures Organotypic cultures with an air–tissue interface were prepared as described [47] . Gels comprised a 50:50 mixture of Matrigel (Becton Dickinson) and type I collagen (Upstate) containing 5 × 10 5 ml −1 of MRC5 cells, to which 5 × 10 5 MDA-468 cells were added on top. For inhibition studies, SU11274 (2 μM) and Gö6976 (1 μM) were added to the MDA-468 growth medium. The medium was changed every 2 days. After 14 days, the gels were bisected, fixed in 4% paraformaldehyde and included in paraffin. Sections (8 μm) were immunostained with the pan-cytokeratin antibody AE1/AE3 (Dako), vimentin (Dako), pan-c-Met (Novocastra), Rac1 (Upstate Biotechnology), Lamp1 (Abcam) and EEA1 (Santa Cruz). To analyse cell invasion, confocal sections were taken randomly through the gels and the distance of migration into the gel from the epithelial layer of the five more migratory colonies per picture measured. Each point on the graph represents the mean between these five colonies and 23 images were analysed per condition. Statistical analyses Two-tailed Student’s t -test was performed, paired between different conditions. Quantitative data are expressed as means±s.e.m. Numbers are the results of at least three independent experiments. For Rac1 PM localization and assessment of membrane ruffles formation (phalloidin), at least 100 cells were counted in each condition for each experiment. Cells were randomly chosen through the field by DAPI detection. One-way analysis of variance test was performed for organotypic cultures. How to cite this article : Ménard, L. et al. Receptor tyrosine kinase c-Met controls the cytoskeleton from different endosomes via different pathways. Nat. Commun. 5:3907 doi: 10.1038/ncomms4907 (2014).